Graphene-contact electrically driven microdisk lasers Active nanophotonic devices are attractive due to their low-power consumption, ultrafast modulation speed and high-density integration. Although electrical operation is required for practical implementation of these devices, it is not straightforward to introduce a proper current path into such a wavelength-scale nanostructure without affecting the optical properties. For example, to demonstrate electrically driven nanolasers, complicated fabrication techniques have been used thus far. Here we report an electrically driven microdisk laser using a transparent graphene electrode. Current is injected efficiently through the graphene sheet covering the top surface of the microdisk cavity, and, for the first time, lasing operation was achieved with a low-threshold current of ~300 μA at room temperature. In addition, we measured significant electroluminescence from a graphene-contact subwavelength-scale single nanopillar structure. This work represents a new paradigm for the practical applications of integrated photonic systems, by conformally mounting graphene on the complex surfaces of non-planar three-dimensional nanostructures. Graphene electronics/photonics have become an emerging research field because of the excellent electrical/optical properties of graphene [1] , [2] . In particular, graphene is promising as a transparent electrode [3] , [4] , [5] because of its high optical transmittance over a broad range of the spectrum spanning visible and infrared (IR) wavelengths, with a theoretical value of 97.7% for monolayer graphene [1] , [6] , as well as remarkably high carrier mobility [7] . Furthermore, graphene, which possesses unusual mechanical strength and elasticity [8] , [9] , can be considered as an alternative to fragile and expensive transparent conducting oxides or thick metals with strong light absorption and scattering properties. Therefore, graphene transparent electrodes have been intensively studied for a broad range of applications, including solar cells [10] , flexible displays [11] , touch screens [3] and organic light-emitting diodes (LEDs) [12] . On the other hand, wavelength-scale nanolasers have been developed, which are promising in that they provide coherent light sources [13] , [14] , [15] , [16] , [17] , and can be combined efficiently with other nanophotonic devices, such as waveguides and detectors, for use in ultracompact photonic integrated circuits [18] , [19] . To take full advantage of these nanolasers, it is desirable to operate them by electrical injection and achieving this is a critical step for realizing most practical applications of photonic systems. However, it is challenging to inject carriers efficiently in a nanophotonic device because the presence of a carrier path near such an ultrasmall cavity tends to seriously disturb the optical properties of the cavity modes. For this reason, previously reported electrically driven nanolasers require complicated fabrication techniques to place submicron-sized electrodes in a desirable position with a subwavelength-scale accuracy [14] , [15] or to construct lateral p–i–n junctions that are aligned well with a nanocavity [13] . Several lasers sacrifice the quality (Q) factors of the resonant modes in a cavity directly contacted to a metal electrode, due to metallic absorption, although the mode volumes were further reduced [16] . In this study, we demonstrate successfully a microdisk laser and a sub-micrometre-sized single nanopillar LED, which are electrically pumped through the transparent and flexible few-layer graphene electrodes. An optically ultrathin graphene sheet combined with a sensibly designed cavity minimizes the optical loss in the cavity and also provides a robust current path. Design and fabrication of graphene-contact microdisk laser The graphene electrode introduced into our laser device has important roles as an efficient carrier spreading layer as well as an electrode for n-type contact, as shown in the schematic diagram of Fig. 1a . Graphene is contacted on the n–i–p microdisk with three InGaAsP quantum wells and the dielectric material outside the microdisk. This outside dielectric material separates the electrically conductive graphene from the p-doped InP substrate. The p-doped central post is placed underneath the microdisk acting as a p-type electrode [14] , [15] . Electrons and holes are then injected through the graphene sheet and central post into the top and bottom layers of the n–i–p microdisk, respectively, and electroluminescence (EL) with a peak wavelength of ~1,550 nm is emitted from the microdisk. In addition, we introduce a dielectric ring structure onto the top of the microdisk, which separates the graphene optically from the boundary of the microdisk, where the whispering-gallery mode (WGM) is highly confined [14] . As few-layer graphene can cause non-negligible optical absorption [20] , the dielectric ring structure will be useful to excite the high-Q WGM in the microdisk cavity with the few-layer graphene electrode. 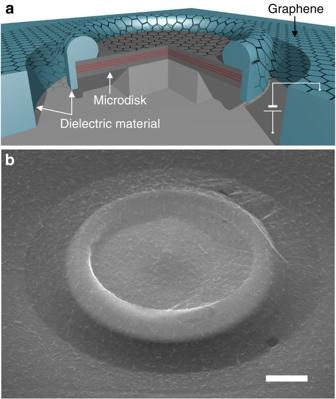Figure 1: Graphene-contact microdisk laser. (a) Schematic diagram (not to scale) of a graphene-contact microdisk laser. A few-layer graphene sheet is mounted onto the microdisk with a dielectric ring structure. The dielectric material outside the microdisk separates electrically conductive graphene from the p-InP substrate. (b) SEM image of a fabricated laser structure. The graphene sheet is freely suspended between the microdisk and the outside dielectric material. The scale bar is 1 μm. Figure 1b shows a scanning electron microscopy (SEM) image of the fabricated graphene-contact microdisk structure. The graphene sheet is well-attached to the surface of the microdisk and suspended freely in air between the microdisk and the outside dielectric material, which is not usually feasible in conventional metal electrodes. Owing to the excellent flexibility and mechanical strength of graphene [8] , [9] , the graphene electrode can be mounted conformally on the complex surface of the non-planar three-dimensional (3D) nanostructure, which has a large height variation of 550 nm from the dielectric ring to the microdisk ( Supplementary Fig. S1h ). Figure 1: Graphene-contact microdisk laser. ( a ) Schematic diagram (not to scale) of a graphene-contact microdisk laser. A few-layer graphene sheet is mounted onto the microdisk with a dielectric ring structure. The dielectric material outside the microdisk separates electrically conductive graphene from the p-InP substrate. ( b ) SEM image of a fabricated laser structure. The graphene sheet is freely suspended between the microdisk and the outside dielectric material. The scale bar is 1 μm. Full size image We fabricated the graphene-contact microdisk structure using the following procedures ( Fig. 2a–d ; Supplementary Fig. S1a–g ). Representative SEM images of the key fabrication steps are shown in Fig. 2a–d . First, a microdisk with a diameter of ~5 μm is fabricated by electron-beam lithography and dry etching, and a dielectric ring structure is fabricated on the top of the microdisk using cross-linked poly(methyl methacrylate) (PMMA), Fig. 2a . Wet etching in diluted hydrochloric acid solution partially removes the InP sacrificial layer underneath the microdisk, which remains as the post structure for the current path ( Fig. 2b ). The dielectric material outside the microdisk is defined by electron-beam lithography, again using cross-linked PMMA ( Fig. 2c ). Finally, the few-layer graphene sheet with the excellent mechanical strength is mounted onto the microdisk and the outside dielectric material ( Fig. 2d ). As all the fabrication steps are straightforward and simple, the yield is high and the fabricated laser structures are reproducible, as shown in the SEM image of large-area array of the microdisk lasers ( Supplementary Fig. S1i ). More detailed procedures are shown in Supplementary Fig. S1a–g . 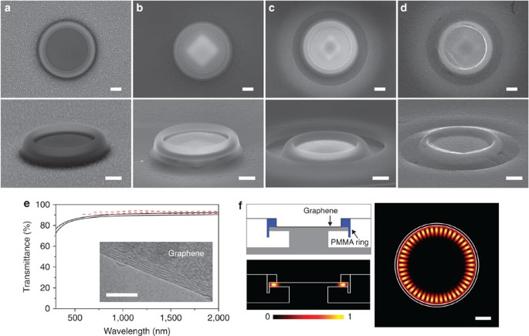Figure 2: Fabrication and optical characterization of the microdisk cavity with few-layer graphene. (a–d) Top (upper panel) and tilted (lower panel) views of the SEM images in each fabrication step. (a) The dielectric ring structure was fabricated onto the microdisk. (b) The wet etching defined the central post underneath the microdisk. (c) The outside dielectric material was fabricated around the microdisk. (d) The graphene sheet was mounted onto the microdisk and the outside dielectric material. The scale bars are all 1 μm. (e) The measured transmittance of graphene sheets with two different thicknesses as a function of wavelength (black solid lines). The calculated transmittance curves of graphene sheets with thicknesses of 1.5 and 2.0 nm are also shown (red dotted lines). The inset shows the transmission electron microscopy image of a representative synthesized graphene sheet with five layers (scale bar, 5 nm). (f) The calculated electric field intensity profiles of the WGM (azimuthal number of 24) in the graphene-contact microdisk cavity with the dielectric ring structure. The Q factor and resonant wavelength were calculated to be 2,100 and 1,550 nm, respectively. The left and right panels show side and top views, respectively, in which electric field intensities were normalized by their maximum values. A graphene thickness of 1.5 nm was used in this simulation. The scale bar in the right panel is 1 μm. Figure 2: Fabrication and optical characterization of the microdisk cavity with few-layer graphene. ( a – d ) Top (upper panel) and tilted (lower panel) views of the SEM images in each fabrication step. ( a ) The dielectric ring structure was fabricated onto the microdisk. ( b ) The wet etching defined the central post underneath the microdisk. ( c ) The outside dielectric material was fabricated around the microdisk. ( d ) The graphene sheet was mounted onto the microdisk and the outside dielectric material. The scale bars are all 1 μm. ( e ) The measured transmittance of graphene sheets with two different thicknesses as a function of wavelength (black solid lines). The calculated transmittance curves of graphene sheets with thicknesses of 1.5 and 2.0 nm are also shown (red dotted lines). The inset shows the transmission electron microscopy image of a representative synthesized graphene sheet with five layers (scale bar, 5 nm). ( f ) The calculated electric field intensity profiles of the WGM (azimuthal number of 24) in the graphene-contact microdisk cavity with the dielectric ring structure. The Q factor and resonant wavelength were calculated to be 2,100 and 1,550 nm, respectively. The left and right panels show side and top views, respectively, in which electric field intensities were normalized by their maximum values. A graphene thickness of 1.5 nm was used in this simulation. The scale bar in the right panel is 1 μm. Full size image Characterization of graphene and numerical simulation To identify the number of graphene sheets used in our devices, transmission electron microscopy analysis (inset, Fig. 2e ) and Raman spectroscopy [21] ( Supplementary Fig. S2 ) were performed. These showed that the synthesized graphene sheet has five to ten layers. In addition, to examine the optical properties of graphene, we measured transmittance as a function of wavelength ( Fig. 2e ). A high transmittance of >91.9% was measured at the peak wavelength of EL (~1,550 nm) and thus the few-layer graphene sheet can be used as a transparent electrode in the near-IR and IR wavelength regions. To quantitatively analyse optical loss in a graphene-contact microdisk cavity, we calculated the transmittance of the graphene sheet and the optical properties of the cavity mode using 3D finite-difference time-domain (FDTD) simulations (Methods and Supplementary Fig. S3 ). It is noted that the calculated transmittance of few-layer graphene sheets with different thicknesses of 1.5 and 2.0 nm (red dotted lines, Fig. 2e ), which correspond to graphene with five-to-seven layers, agrees well with the experimental results (black solid lines, Fig. 2e ). We also calculated the mode profiles and Q factor of the microdisk topped with 1.5-nm-thick graphene, using the structural parameters taken from SEM images of the fabricated device ( Fig. 2f ). The WGM is well-excited in the graphene-contact microdisk and the electric field is strongly confined at the boundary of the microdisk. As the dielectric ring structure introduced on the top of the microdisk minimizes the optical loss by graphene, a high Q factor of ~2,100 was calculated. This value is ~12 times higher than the calculated Q factor without the dielectric ring structure, which was 170 ( Supplementary Fig. S3d ). Therefore, the rational cavity design including the dielectric ring structure will be highly useful to avoid undesired absorption loss by few-layer graphene and demonstrate a low-threshold lasing operation. Measurement of lasing properties The fabricated microdisk cavity was electrically pumped by using 100 ns current pulses for a period of 1 μs at room temperature. Current was injected using a metal tip, which was contacted the graphene on the dielectric material outside the microdisk ( Supplementary Fig. S1j ). The light emitted from the microdisk was collected by a ×20 or ×50 long-working-distance microscope objective lens focused onto either a spectrometer or an IR camera (see Methods ). As the injected current increased, a sharp, dominant peak was detected along with a rapid increase in intensity. At the further increased current, single-mode lasing was observed at a wavelength of 1,540.5 nm, as shown in Fig. 3a . In addition, the lasing mode image captured by the IR camera shows strong light emission at the boundary of the microdisk cavity (inset, Fig. 3a ). 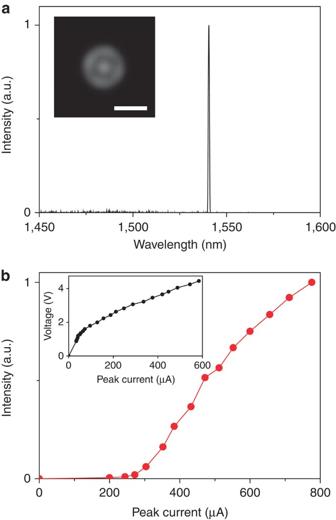Figure 3: Electrically driven microdisk laser. (a) Above-threshold lasing spectrum measured at a peak current of 810 μA. Pulsed current with a 10% duty cycle was injected. Single-mode lasing was observed at a wavelength of 1,540.5 nm. The inset shows the lasing mode image captured by an IR camera at a current of 700 μA (scale bar, 5 μm). (b) Measured lasing intensity as a function of the injected peak current. The threshold current is ~300 μA. The inset shows the current–voltage characteristics of the laser device. Figure 3: Electrically driven microdisk laser. ( a ) Above-threshold lasing spectrum measured at a peak current of 810 μA. Pulsed current with a 10% duty cycle was injected. Single-mode lasing was observed at a wavelength of 1,540.5 nm. The inset shows the lasing mode image captured by an IR camera at a current of 700 μA (scale bar, 5 μm). ( b ) Measured lasing intensity as a function of the injected peak current. The threshold current is ~300 μA. The inset shows the current–voltage characteristics of the laser device. Full size image To clearly measure the transition to the lasing mode, we measured the output intensity of the mode as a function of the injected peak current ( Fig. 3b ). In this plot, a superlinear increase in output intensity can be clearly observed at a low-lasing threshold of ~300 μA. This threshold current is comparable with those of the previously reported microdisk lasers of similar size [14] , [18] , [19] . Analysis of the linewidth as a function of injected current showed a decrease in linewidth to the resolution limit of the spectrometer, ~0.75 nm, as the injected current increases from below to above the threshold current. In this case, the experimental Q factor of the cavity can be estimated to be >2,100, which agrees well with the FDTD simulation result obtained in Fig. 2f . In addition, the electrical properties of the microdisk laser are shown by the voltage versus current curve (inset, Fig. 3b ). The turn-on voltage and electrical resistance are ~1.2 V and ~5.8 kΩ, respectively. The relatively high resistance is mainly caused by the contact resistance between the graphene and the InGaAsP material of the microdisk, because the contact resistance is estimated to be ~4.9 kΩ from the result of the transmission line method measurement [8] ( Supplementary Fig. S4a ). This contact resistance can be reduced significantly by introducing a metal layer between the graphene contact and semiconductor material [8] , [22] . Indeed, we measured a low device resistance of ~2.3 kΩ using a graphene top contact with a gold layer on the central region of the microdisk ( Supplementary Fig. S5 ). The contact resistance can also be reduced by increasing the doping of the semiconductor or graphene [23] , [24] . On the other hand, we note that the graphene contact provides efficient current spreading and uniform current injection into the n-InGaAsP epilayer of the microdisk due to the low sheet resistance of graphene ( Supplementary Fig. S4b,c ). We changed the injected current pulse width from 100 to 500 ns for a period of 1 μs to examine the possibility of continuous-wave (CW) lasing operation. Lasing operation was achieved by injection of current pulses with ≤30% duty cycles and showed almost identical threshold currents and lasing wavelengths for each pulse width ( Supplementary Fig. S6 ). However, we could not observe lasing when using a current pulse with a 50% duty cycle, for which significant red shift of the wavelength and linewidth broadening occurred. These observations indicate that the injection of a broad pulse with a >50% duty cycle can cause a significant heat problem in the microdisk with few-layer graphene. Compared with a conventional microdisk cavity with a similar-sized post structure enabling CW lasing operation [14] , [25] , the relatively high contact resistance could be a major origin of this thermal issue in the graphene-contact microdisk. In contrast, we measured improved lasing properties from the graphene-contact microdisk laser with a thin gold layer on the central region of the microdisk ( Supplementary Fig. S7 ). Owing to the reduced resistance in this device, lasing operation was successfully achieved by injection of a broad current pulse with a 50% duty cycle. We believe that further improvement of our laser device to reduce the contact resistance will allow us to demonstrate CW lasing operation. Graphene-contact single nanopillar LED To take full advantage of the transparent graphene electrode, we carried out electrical pumping in a submicrometer-sized single nanopillar LED. A few-layer graphene sheet was introduced onto a nanopillar structure with a diameter of <500 nm, without the dielectric ring and post structures, as shown in the SEM image of Fig. 4a . The white dotted line indicates the boundary of the dielectric material outside the nanopillar (inset, Fig. 4a ). The observed bright spot of the mode image shows significant light emission from the nanopillar (inset, Fig. 4b ). The EL spectrum with a peak wavelength of ~1,600 nm was also clearly measured ( Fig. 4b ). These measurements show that in spite of an ultrasmall size of the nanopillar, the graphene electrode injects current efficiently into the single nanopillar LED. The remarkable demonstration of an electrically driven single nanopillar LED suggests the feasibility of efficient electrical pumping into various nanophotonic devices such as plasmonic lasers [26] , [27] , nanowire lasers [17] and micro/nanopillar devices [28] , [29] . 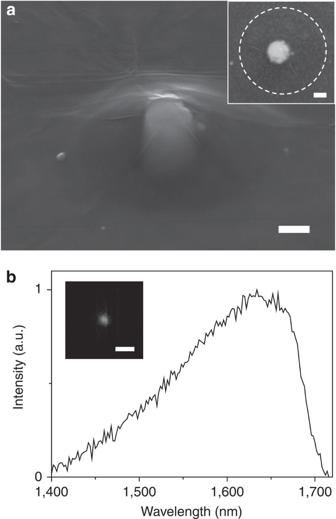Figure 4: Submicrometre-sized single nanopillar LED with few-layer graphene. (a) SEM image of a nanopillar LED with a transparent graphene electrode. The scale bar is 300 nm. The inset shows the top view of the structure, where the white dotted line indicates the boundary of the dielectric material outside the nanopillar (scale bar, 300 nm). Dielectric ring and post structures were not fabricated. (b) Measured EL spectrum of the single nanopillar LED at a current of 1,800 μA. The inset shows the EL image captured by an IR camera at 1,500 μA. Pulsed current with a 5% duty cycle was injected. The scale bar is 5 μm. Figure 4: Submicrometre-sized single nanopillar LED with few-layer graphene. ( a ) SEM image of a nanopillar LED with a transparent graphene electrode. The scale bar is 300 nm. The inset shows the top view of the structure, where the white dotted line indicates the boundary of the dielectric material outside the nanopillar (scale bar, 300 nm). Dielectric ring and post structures were not fabricated. ( b ) Measured EL spectrum of the single nanopillar LED at a current of 1,800 μA. The inset shows the EL image captured by an IR camera at 1,500 μA. Pulsed current with a 5% duty cycle was injected. The scale bar is 5 μm. Full size image We successfully demonstrated electrically driven microdisk lasers and subwavelength-scale single nanopillar LEDs using a transparent graphene electrode at room temperature. The graphene electrode, which contacts conformally over the complicated nanostructured surfaces and is also freely suspended in air, is unique and distinguishable from the conventionally used metal electrodes. The use of graphene as a transparent electrode will enrich the applications of graphene in nanophotonic devices and open a new paradigm for the practical applications of ultracompact photonic integrated systems. Graphene synthesis Large-area, few-layer graphene films were synthesized using a home-built chemical vapour deposition system that consists of a horizontal tube furnace [8] . First, a 200-nm-thick Ni film was deposited on a 200-nm-thick SiO 2 /Si substrate using a thermal evaporator, and this sample was transferred to the quartz tube reactor. The reactor was evacuated to a pressure well <100 mTorr and filled again with an H 2 /Ar gas mixture (25% H 2 in Ar) until the pressure reached atmospheric pressure. The Ni/SiO 2 /Si substrate was then annealed at 1,000 °C for 30 min under a H 2 and Ar gas mixture at a flow rate of 60 sccm, followed by turning on the flow of methane gas (10 sccm). After resting the sample for 1 min, the methane gas supply was terminated and the chamber was quickly cooled down to room temperature with a cooling rate of ~10 °C s −1 under a continuous H 2 and Ar atmosphere. During cooling, carbon atoms were segregated from the Ni film, resulting in the formation of a few-layer graphene sheet. The synthesized graphene film was coated with a thin protecting layer of PMMA. By submerging the sample in an HF solution, the Ni and SiO 2 layers were etched and the PMMA/graphene sheet was separated from the substrate. The remaining Ni layer underneath the PMMA/graphene sheet was additionally removed by an aqueous Ni etchant, TFG, followed by rinsing with water. Then, the hydrophobic PMMA/graphene sheets floated on the water and could be easily moved onto various substrates such as a transmission electron microscopy grid or glass, for structural and optical characterization. Device fabrication Microdisk or nanopillar structures were fabricated using (260-nm-thick n–i–p InGaAsP slab)/(1-μm-thick p-InP sacrificial layer)/(p-InP substrate) wafer structure. Three layers of InGaAsP quantum wells are embedded in the slab. The fabrication procedure of the graphene-based cavity structure is shown in detail in Supplementary Fig. S1a–g . EL measurement The EL from the graphene-contact microdisk or nanopillar cavity was measured at room temperature by contacting a tungsten tip with a diameter of 1 μm to the graphene sheet mounted on the dielectric material outside the cavity. The sample was attached to an aluminium plate using a conductive silver paste. The forward bias was applied from the aluminium plate to the tungsten tip. We used a pulse generator (Agilent 33521A) and changed the pulse width for a period of 1 μs. The light emitted from the individual microdisk or nanopillar was collected by an ×20 long-working-distance objective lens (with a numerical aperture of 0.4) focused onto either a spectrometer with a resolution limit of ~0.75 nm or an InGaAs IR charge-coupled device camera. The mode image in Fig. 3a was captured by an IR camera using a ×50 long-working-distance objective lens with a numerical aperture of 0.42. FDTD calculations In the 3D FDTD simulation, refractive indices of graphite were used to represent few-layer graphene sheets. The graphite was modelled by the Drude critical points (D-CP) model, which can model dispersive material over a wide spectrum [30] , [31] : where in which is the background dielectric constant at infinite frequency, ω is the angular frequency, ω D and ω p are the electron plasma frequencies, γ D and γ p are the effective collision frequencies, φ p is the phase, A p is the weighting coefficient and p is number of critical poles. The D-CP model fits the experimentally determined dielectric functions of graphite in the near-IR and visible spectral range (0.2–1.4 eV) (ref. 32 ) [32] . Parameters used in our simulations were as follows: =4.53, ω D =8.31 eV, γ D =10.86 eV, ω p 1 =1.07, γ p 1 =0.17 eV, A p 1 =−0.53, φ p 1 =0.078 rad, ω p 2 =0.30 eV, γ p 2 =0.35 eV, A p 2 =−10.28, φ p 2 =0.99 rad, where two critical poles were assumed. The D-CP model with the parameters for graphite fits the experimental measured refractive indices over a broad range of spectrum as shown in Supplementary Fig. S3b . To represent nanometer-scale graphene sheets, vertical mesh size of 0.5 nm was used. Because of a relatively large horizontal size of microdisk, horizontal mesh size of 10 nm was used to save computational memory. The refractive indices of the InGaAsP microdisk and the PMMA layer were set to 3.4 and 1.5, respectively, in the 3D FDTD simulation. The uniaxial perfectly matched layer was used for the appropriate absorbing boundary condition [33] . How to cite this article: Kim, Y.-H. et al . Graphene-contact electrically driven microdisk lasers. Nat. Commun. 3:1123 doi: 10.1038/ncomms2137 (2012).